Catch rate composition affects assessment of protected area impacts 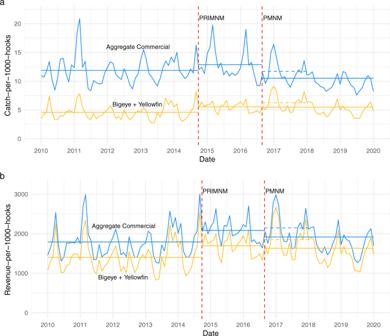Fig. 1: Monthly CPUE and RPUE calculated using two measures of catch composition. aCatch-per-1000-hooks measured by aggregate commercial catch (blue) and Bigeye + Yellowfin tuna catch (gold) calculated using data from the NOAA Observer Program. Solid horizontal lines indicate average catch rates over the designated time periods. Dashed lines indicate average catch rates in the post-PMNM expansion period presented in Lynham et al.1. The two red dashed lines indicate the Pacific Remote Island Marine National Monument expansion (PRIMNM) and the Papahānaumokuākea Marine National Monument expansion (PMNM).bRevenue-per-1000-hooks aggregated for 11 commercially caught species (blue) and Bigeye +  Yellowfin (gold). Revenue-per-1000-hooks was approximated by multiplying the number of individuals caught by the average value of individual fish for each species, then dividing by effort measured in 1000 s of hooks. The average value of individual fish was calculated using observed fish sales from 2010 to 2019 from Hawaii’s dealer data. The two red dashed lines indicate the Pacific Remote Island Marine National Monument expansion (PRIMNM) and the Papahānaumokuākea Marine National Monument expansion (PMNM). 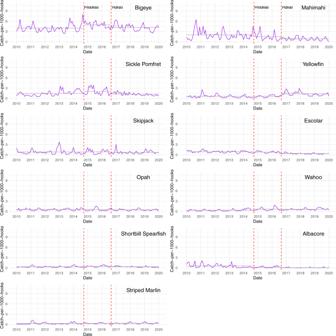Fig. 2: Monthly CPUE for 11 commercial species caught in Hawaii’s deep-set longline fishery. Catch-per-1000-hooks for 11 commercially caught species in Hawaii’s deep-set longline fishery calculated using data from the NOAA Observer Program. Solid grey lines indicate average catch rates over the designated time periods. Dashed grey lines indicate average catch rates in the post-PMNM expansion period presented in Lynham et al.1. The two red dashed lines indicate the Pacific Remote Island Marine National Monument expansion (PRIMNM) and the Papahānaumokuākea Marine National Monument expansion (PMNM). Further information on research design is available in the Nature Research Reporting Summary linked to this article.